Hydrodynamic phonon transport in suspended graphene Recent studies of thermal transport in nanomaterials have demonstrated the breakdown of Fourier’s law through observations of ballistic transport. Despite its unique features, another instance of the breakdown of Fourier’s law, hydrodynamic phonon transport, has drawn less attention because it has been observed only at extremely low temperatures and narrow temperature ranges in bulk materials. Here, we predict on the basis of first-principles calculations that the hydrodynamic phonon transport can occur in suspended graphene at significantly higher temperatures and wider temperature ranges than in bulk materials. The hydrodynamic transport is demonstrated through drift motion of phonons, phonon Poiseuille flow and second sound. The significant hydrodynamic phonon transport in graphene is associated with graphene’s two-dimensional features. This work opens a new avenue for understanding and manipulating heat flow in two-dimensional materials. The transport of phonons, which are the dominant heat carriers in non-metallic solids, is usually diffusive and describable by Fourier’s law of heat conduction. Regimes where Fourier’s law breaks down, such as ballistic [1] and hydrodynamic [2] phonon transport, were discovered in bulk materials more than 50 years ago, but these phenomena were observed only at extremely low temperatures [3] , [4] , [5] . Recent studies of low-dimensional materials, however, have highlighted the practical importance of ballistic phonon transport in applications such as thermoelectric materials [6] and electronic devices [7] , [8] . In this work, we discuss how hydrodynamic phonon transport as well as ballistic phonon transport can be significant in a two-dimensional material, particularly in graphene. The term hydrodynamic phonon transport arose from its similarity with macroscopic transport phenomena in fluids. In fluid flow, mass transport is mainly due to the macroscopic motion of molecules with a drift velocity. Likewise, phonons in the hydrodynamic regime exhibit macroscopic drift motion. In this sense, hydrodynamic phonon transport is different from the more well-known diffusive or ballistic phonon transport. During diffusive transport, heat is transferred through multiple scattering events among phonons without macroscopic drift motion. During ballistic transport, it is assumed that there is no internal scattering. Hydrodynamic transport, on the other hand, includes many phonon scattering events. The drift motion of phonons in the hydrodynamic regime causes two interesting hydrodynamic transport phenomena that cannot occur in either diffusive or ballistic regimes: phonon Poiseuille flow ( Fig. 1a ) and second sound ( Fig. 1c ), which are analogous to Poiseuille flow and ordinary sound in a fluid, respectively, which will be discussed later. 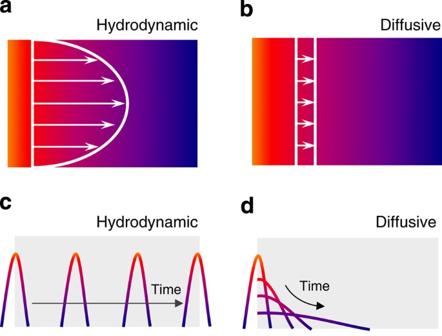Figure 1: The different macroscopic transport phenomena in hydrodynamic and diffusive regimes. (a,b) The steady-state heat flux profiles in hydrodynamic and ballistic regimes, respectively, under a temperature gradient. (a) Phonons in the hydrodynamic regime exhibit a non-uniform heat flux profile like the mass flux profile of fluid flow in a tube. In the hydrodynamic regime, the main mechanism for momentum loss is diffuse boundary scattering. Therefore, the flux is small near the boundary. (b) In the diffusive regime, however, the heat flux profile has a uniform shape. This is because transport resistance is mainly due to intrinsic momentum loss scattering called Umklapp scattering rather than diffuse boundary scattering. The Umklapp scattering can occur anywhere inside a sample, leading to a uniform heat flux profile. (c,d) The propagation of a heat pulse in the hydrodynamic and diffusive regimes, respectively. (c) In the hydrodynamic regime, a heat pulse propagates like a pressure pulse (ordinary sound) in a fluid without significant damping. The invoked pulse can transmit through the sample and finally arrive at the edge of the sample with well-preserved pulse shape. (d) In the diffusive regime, however, a heat pulse is significantly damped and cannot propagate. The pulse smears out and reaches the edge of the sample after a relatively long time. The width and length of the sample are assumed to be much larger than the phonon mean free path. Figure 1: The different macroscopic transport phenomena in hydrodynamic and diffusive regimes. ( a , b ) The steady-state heat flux profiles in hydrodynamic and ballistic regimes, respectively, under a temperature gradient. ( a ) Phonons in the hydrodynamic regime exhibit a non-uniform heat flux profile like the mass flux profile of fluid flow in a tube. In the hydrodynamic regime, the main mechanism for momentum loss is diffuse boundary scattering. Therefore, the flux is small near the boundary. ( b ) In the diffusive regime, however, the heat flux profile has a uniform shape. This is because transport resistance is mainly due to intrinsic momentum loss scattering called Umklapp scattering rather than diffuse boundary scattering. The Umklapp scattering can occur anywhere inside a sample, leading to a uniform heat flux profile. ( c , d ) The propagation of a heat pulse in the hydrodynamic and diffusive regimes, respectively. ( c ) In the hydrodynamic regime, a heat pulse propagates like a pressure pulse (ordinary sound) in a fluid without significant damping. The invoked pulse can transmit through the sample and finally arrive at the edge of the sample with well-preserved pulse shape. ( d ) In the diffusive regime, however, a heat pulse is significantly damped and cannot propagate. The pulse smears out and reaches the edge of the sample after a relatively long time. The width and length of the sample are assumed to be much larger than the phonon mean free path. Full size image Despite the interesting features of hydrodynamic phonon transport, the temperature range in which it was observed was too low and narrow to consider for practical applications. For example, the reported temperature range for phonon Poiseuille flow is 0.5–1.0 K (ref. 5 ) and for second sound the range is 10–20 K (ref. 9 ). The extremely stringent temperature conditions for hydrodynamic phonon transport are due to Umklapp scattering (hereafter U-scattering), which destroys the crystal momentum. In contrast, scatterings between molecules conserve total momentum. As such, for hydrodynamic transport to occur, U-scattering should be negligibly weak compared with the other three-phonon scattering, which conserves crystal momentum, normal scattering (hereafter N-scattering). One way to suppress U-scattering is to consider low temperatures, but at too low temperatures transport becomes ballistic without internal scattering, leaving only a very narrow temperature range for hydrodynamic transport. In addition to U-scattering, the scattering of phonons by impurities such as isotopes does not conserve crystal momentum, and isotope enrichment imposes another difficulty for hydrodynamic phonon transport (hereafter R-scattering denotes Umklapp and isotope scatterings). Here, we show that suspended graphene (hereafter graphene), unlike three-dimensional materials, is remarkably well suited for hydrodynamic phonon transport. Using first-principles calculations, we show drift motion of phonons, phonon Poiseuille flow and second sound in graphene at significantly higher and wider temperature ranges compared with those seen in three-dimensional materials. Then, we discuss how the significant hydrodynamic phonon transport in graphene stems from its two-dimensional features. Displaced distribution function An indication of the hydrodynamic transport, the macroscopic drift motion, can be found in the distribution function. For example, for molecules in fluid flow, the Maxwell distribution displaced by a drift velocity is considered an equilibrium distribution [10] . Similarly, if there is no R-scattering among phonons, the displaced Bose–Einstein distribution has been commonly assumed for the equilibrium distribution of phonons [11] . where ħ , ω and q represent the Planck constant, phonon frequency and phonon wavevector, respectively. The drift velocity is represented by the displacement, u , in the phonon distribution. In the displaced distribution, the displacement is a constant for all phonon modes regardless of polarization and wavevector, describing the macroscopic drift motion of phonons having the same velocity. Assuming a small drift velocity, this displaced distribution can be linearized to where is the Bose–Einstein distribution. On the basis of the assumption of the displaced phonon distribution in the absence of R-scattering, past work derived macroscopic governing equations that describe hydrodynamic phonon transport [12] . However, it has remained elusive to our knowledge whether the absence of R-scattering necessarily leads to the displaced distribution. Moreover, the validity of the displaced distribution in real materials, where R-scattering cannot be completely avoided, has not been explicitly confirmed. In this work, we demonstrate from first-principles calculations that a displaced distribution of phonons can occur in graphene even in the presence of weak R-scattering, which validates the assumption of the displaced distribution used in the past studies [12] , [13] and correspondingly shows hydrodynamic phonon transport in graphene. The recent progress in calculating the phonon–phonon scattering matrix using first-principles [14] , [15] and numerical methods for solving the Peierls–Boltzmann equation [16] , [17] enable the calculation of phonon distributions in a specific material under a temperature gradient. This first principles-based method has been demonstrated to be highly accurate and have predictive power for phonon transport in many materials including graphene [15] , [18] , [19] , [20] , [21] , [22] , [23] . In this work, to capture the significant role of N-scattering, we solve the full solution of the Peierls–Boltzmann equation without relaxation time approximation. In Fig. 2 , we show this phonon distribution in an infinitely large graphene sheet with 0.1% concentration of isotope 13 C at 100 K under a static temperature gradient. The temperature gradient is required to maintain the drift motion since R-scattering cannot be completely ignored in real materials. 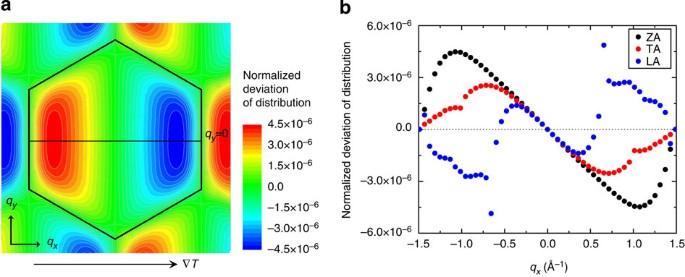Figure 2: The displaced distribution of phonons at 100 K in reciprocal space of a graphene sheet. The13C isotope concentration is 0.1%. (a) A contour plot of the normalized deviation of distribution,, of flexural acoustic (ZA) phonons in graphene. The hexagon represents the first Brillouin zone and a temperature gradient is applied along thexdirection. (b) The normalized deviation of distribution of the three acoustic branches in graphene along thexdirection atqy=0 (M–Γ–M). The linear dependence onqxindicates drift motion of acoustic modes, according to equation (2). The same slope for all three acoustic branches means acoustic phonons have the same drift velocity regardless of polarization and wavevector. Figure 2 plots the normalized deviation of the distribution from the stationary equilibrium distribution, defined as , to examine the existence of a drift velocity. It is clearly seen in Fig. 2b that the normalized deviation is linear to wavevector q x along the temperature gradient direction with the same slope for all three acoustic branches in a wide range of wavevectors. This indicates that the distribution is indeed displaced, giving the macroscopic motion of phonons with the same velocity as in equation (2). In usual cases without strong hydrodynamic transport features, the normalized deviation shows no correlation among phonon modes and phonons cannot exhibit any macroscopic collective motion (see Supplementary Note 1 and Supplementary Fig. 3 for an example) The non-linear behaviour in the large wavevector region of Fig. 2b is significantly exaggerated because the deviation is normalized by , which is negligibly small in this high phonon frequency range. Moreover, these phonon modes in the range where the normalized deviation is non-linear to q x contribute negligibly to actual thermal transport. (See Supplementary Fig. 1 ) Figure 2: The displaced distribution of phonons at 100 K in reciprocal space of a graphene sheet. The 13 C isotope concentration is 0.1%. ( a ) A contour plot of the normalized deviation of distribution, , of flexural acoustic (ZA) phonons in graphene. The hexagon represents the first Brillouin zone and a temperature gradient is applied along the x direction. ( b ) The normalized deviation of distribution of the three acoustic branches in graphene along the x direction at q y =0 (M–Γ–M). The linear dependence on q x indicates drift motion of acoustic modes, according to equation (2). The same slope for all three acoustic branches means acoustic phonons have the same drift velocity regardless of polarization and wavevector. Full size image The macroscopic drift motion of phonons can be explained by strong N-scattering compared with R-scattering shown in Fig. 3b . The phonon distribution under a temperature gradient is slightly displaced, meaning that the phonons gain excess momentum from the temperature gradient. Then, the excess momentum is affected by N- and R-scatterings in very different ways [24] . Through N-scatterings, the excess momentum is exchanged among phonons such that all phonon modes exhibit the same drift velocity and approach the displaced Bose–Einstein distribution in equation (1). However, R-scattering destroys the excess momentum and induces phonon modes to relax to the stationary equilibrium Bose–Einstein distribution. In graphene, N-scattering is much stronger than R-scattering by at least two orders of magnitude in a wide spectrum as shown in Fig. 3b . Therefore, the excess momentum gained from a temperature gradient is redistributed by strong N-scattering without any considerable reduction by R-scattering such that most phonon modes have the same drift velocity regardless of polarization and wavevector. 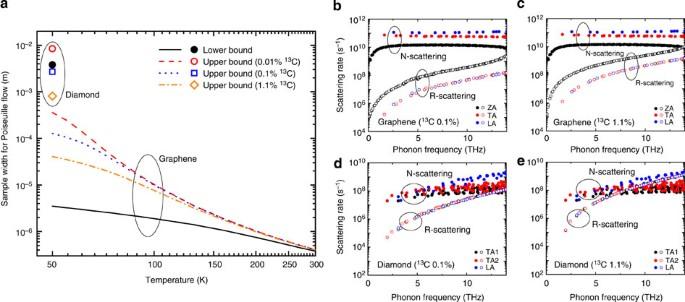Figure 3: The wide window of sample widths for phonon Poiseuille flow in graphene due to strong N-scattering. (a) The upper and lower bounds of sample width for phonon Poiseuille flow in graphene and diamond. The lower bound is set to prevent ballistic transport. The upper bound is required so that momentum loss by diffuse boundary scattering combined with N-scattering is stronger than that by R-scattering. Graphene has a wide gap between the lower and upper bounds below 100 K, indicating that phonon Poiseuille flow can occur in the corresponding temperature range. Diamond, however, has a negligibly small gap even at 50 K with extremely enriched isotope content, 0.01%13C. (b–e) Comparison between N- and R-scattering rates in graphene and diamond at 100 K, showing extremely strong N-scattering in graphene. The condition of isotope content is specified in the plots. The isotope content of 1.1%13C in (c,e) represents the naturally occurring case. Figure 3: The wide window of sample widths for phonon Poiseuille flow in graphene due to strong N-scattering. ( a ) The upper and lower bounds of sample width for phonon Poiseuille flow in graphene and diamond. The lower bound is set to prevent ballistic transport. The upper bound is required so that momentum loss by diffuse boundary scattering combined with N-scattering is stronger than that by R-scattering. Graphene has a wide gap between the lower and upper bounds below 100 K, indicating that phonon Poiseuille flow can occur in the corresponding temperature range. Diamond, however, has a negligibly small gap even at 50 K with extremely enriched isotope content, 0.01% 13 C. ( b – e ) Comparison between N- and R-scattering rates in graphene and diamond at 100 K, showing extremely strong N-scattering in graphene. The condition of isotope content is specified in the plots. The isotope content of 1.1% 13 C in ( c , e ) represents the naturally occurring case. Full size image In addition to the macroscopic collective motion of phonons, it is also important to find the specific length and timescales for hydrodynamic transport. If length and timescales approach infinity, the transport is not hydrodynamic unless R-scattering is completely avoided. Owing to the existence of R-scattering, as we previously stated, a temperature gradient is required to maintain the drift motion of phonons in Fig. 2 . In an infinitely large graphene sheet under a static temperature gradient, the drift velocity of phonons exhibits a uniform distribution across the sample and its magnitude scales as the magnitude of the temperature gradient, both of which can be explained by Fourier’s law. However, roughly speaking, if the sample size is smaller than the phonon mean free path of R-scattering or the temperature gradient changes with time faster than the R-scattering rate, the transport cannot be described by the diffusive law. In such length and timescales, the transport with macroscopic drift motion shown in Fig. 2 can be hydrodynamic. These considerations regarding length and timescales for hydrodynamic transport lead to the discussion on phonon Poiseuille flow and second sound in the following sections. The displaced distribution we present here is the first explicit confirmation of the assumption used in past theoretical studies regarding hydrodynamic phonon transport [12] , [13] , [25] , [26] . It also provides a theoretical basis that we will exploit to examine phonon Poiseuille flow and second sound in the following sections, further highlighting the significant hydrodynamic phonon transport in graphene. Phonon Poiseuille flow Phonon Poiseuille flow refers to the steady-state hydrodynamic phonon transport under a temperature gradient in a sample. The temperature gradient plays a similar role as pressure gradient for the molecular Poiseuille flow. Here it is assumed that the sample is long enough for the heat flux to be fully developed and to be invariant along the flow direction. Owing to their differing sources of thermal resistance, phonon Poiseuille flow is distinctly different from the more well-known diffusive phonon transport. In diffusive phonon transport, thermal resistance is mostly due to R-scattering, which can occur anywhere inside a sample. Therefore, the heat flux in diffusive phonon transport is uniform, as shown in Fig. 1b . On the other hand, the thermal resistance in phonon Poiseuille flow is due to diffuse boundary scattering combined with many N-scatterings, analogous to viscous effects in fluid flow. The drift velocity is small near the boundary because of diffuse boundary scattering, leading to the formation of a drift velocity gradient along the direction perpendicular to heat flow ( Fig. 1a ). The boundary scattering can be assumed to be diffuse rather than specular even at low temperature such as 100 K. (see Supplementary Fig. 4 and Supplementary Note 2 .) The excess momentum of phonons from the temperature gradient is then transferred to the boundary through the drift velocity gradient and many N-scattering events, and finally destroyed by diffuse boundary scattering. Therefore, thermal conductivity largely depends on the rate of momentum transfer to the boundary, a quantity that is determined by N-scattering rates and a sample width, just as resistance in fluid flow depends on viscosity and a pipe diameter. The significance of the extrinsic momentum loss mechanism in the hydrodynamic regime, diffuse boundary scattering, implies that a material’s thermal conductivity largely depends on the sample shape and geometry in contrast to the diffusive case. This is also much different from the ballistic case since the sample size in the hydrodynamic regime is assumed to be much larger than phonon mean free path. The momentum loss mechanism in phonon Poiseuille flow imposes constraints on sample width in order for phonon Poiseuille flow to occur [26] . If the width of a sample is too large, the excess momentum is more likely to be destroyed by R-scattering before being transferred to the boundary. In this case, the transport is close to the diffusive regime rather than the hydrodynamic regime. On the other hand, if the sample width is less than the phonon mean free path, transport is ballistic. These considerations determine the upper and the lower bounds, respectively, of the sample width for phonon Poiseuille flow (see Methods and Supplementary Note 3 for details). A window of sample widths for phonon Poiseuille flow, calculated from first principles, is shown in Fig. 3a . We also present the results for another allotrope of carbon, diamond, for comparison with graphene, since diamond features weak U-scattering compared with N-scattering owing to its large Debye temperature [27] , [28] . The figure shows that graphene has a much wider window of sample widths for phonon Poiseuille flow than diamond. The possible range of sample widths in diamond with an extremely enriched isotope content (0.01% 13 C) is too narrow even at the lowest temperature we examined (50 K). With a moderately enriched isotope condition (0.1% 13 C), there is no possible sample width for which phonon Poiseuille flow would occur. The results for diamond confirm the significant difficulty in observing hydrodynamic phonon transport in three-dimensional materials [5] . In graphene, however, there is a large window of sample widths at temperatures below 100 K. When the isotope content is increased from 0.01 to 0.1%, the window becomes narrower but is still very wide at temperatures below 100 K. Graphene’s exceptionally wide range of temperatures and sample widths for phonon Poiseuille flow is due to the strong N-scattering shown in Fig. 3b . We compare the scattering rates of graphene and diamond in ( Fig. 3b–e ) to highlight the strong N-scattering in graphene. The N-scattering rates in graphene are around 10 10 s −1 , whereas in diamond they are 10 8 s −1 at 100 K. Owing to the strong N-scattering in graphene, R-scattering remains comparatively small even when the isotope content matches the naturally occurring case, 1.1% 13 C ( Fig. 3c ). In diamond, however, R-scattering rates are comparable to N-scattering rates at the same isotope content ( Fig. 3e ). The underlying reasons for the strong N-scattering in graphene will be further discussed later. For the experimental confirmation of phonon Poiseuille flow, thermal conductivity can be measured by varying sample width. Here we briefly discuss several transport regimes in various sample widths. When the sample width is much larger than the mean free path of R-scattering, transport is diffusive and thermal conductivity does not vary with sample width. As the sample width decreases such that it is smaller than the mean free path of R-scattering but larger than the mean free path of N-scattering, the phonon transport can be described by Poiseuille flow. It is well known that the mass flow rate of molecular Poiseuille flow in two-dimensional duct scales as the third power of duct width. Similarly, in phonon Poiseuille flow, heat flow rate and thermal conductivity scale as the third power and the second power of sample width, respectively. (see Supplementary Note 4 and Supplementary Fig. 7 for details) The thermal conductivity that is superlinearly proportional to sample width makes phonon Poiseuille flow distinguished from the diffusive transport. As the sample width is further decreased and comparable to the mean free path of N-scattering, the transport regime is in between hydrodynamic and ballistic limits. In this case, the phonon system is similar to rarefied gas in a molecule system and it may be possible to observe phonon Knudsen minimum [29] . The phonon Knudsen minimum was observed in liquid helium where phonons carry most of heat at extremely low temperature [30] , [31] . If the sample width is further decreased and much smaller than the phonon mean free path of N-scattering, the transport is ballistic. The thermal conductivity in the ballistic regime described by the Casimir limit cannot be superlinearly proportional to the sample width. The thermal conductivity should be always sublinearly or linearly proportional to the sample width. Therefore, the superlinear dependence of thermal conductivity on sample width can be used for confirming phonon Poiseuille flow. However, there are several possible challenges in actual experiments. For example, one may need several graphene samples that have different sample widths but have the same quality in terms of isotope content or other defect density. The possible variations in the quality between several samples can make it untrustworthy to deduce any trend of thermal conductivity as a function of sample width. In addition, the superlinear dependence of thermal conductivity on sample width may not be a decisive evidence for hydrodynamic transport. The superlinear dependence was also observed in ballistic transport regime in silicon nanowires with roughened surface [32] . Another indication of phonon Poiseuille flow, which has been used in the past work [5] , [33] , [34] , is found in how thermal conductivity changes with temperature. An increase in the thermal conductivity with an exponent in temperature larger than that for the ballistic case is regarded as a direct evidence of phonon Poiseuille flow [26] , [35] . In the ballistic regime, thermal conductivity, κ , can be expressed with a simple formula, κ ~ cvL , where c is a specific heat, v is a group velocity and L is a characteristic size of sample limiting phonon mean free path. Since the sample size, L , is not changed with temperature, an increase of thermal conductivity with temperature should be associated only with specific heat and group velocity, both together determining thermal conductance in the ballistic limit. In the hydrodynamic regime, however, the effective sample size for the boundary scattering increases with temperature. This is because the N-scattering rate increases with temperature, leading to a longer travel distance of phonons to the boundary as discussed in Supplementary Note 3 . The effective sample size for boundary scattering as well as the ballistic thermal conductance, cv , increase with temperature. Therefore, the thermal conductivity in the hydrodynamic regime should increase more rapidly than the ballistic thermal conductance increases with temperature. Considering that the thermal conductance of graphene in the ballistic limit increases as T 1.68 (ref. 36 ), an observation of the thermal conductivity increasing with an exponent in temperature much larger than 1.68 can indicate phonon Poiseuille flow. In recent years, there have been many successful measurements of the thermal conductivity of graphene, but more advances would be required to observe phonon Poiseuille flow. For thermal conductivity measurements using Raman spectroscopy, the temperature range was limited to temperatures above room temperature because of large uncertainties near room temperature [37] , [38] , [39] , [40] . Alternatively, a microfabricated heater-sensor-assembly was used [41] , [42] , [43] , but the samples were not isotopically enriched and too small to observe phonon Poiseuille flow. Second sound Second sound refers to the propagation of a temperature wave (or phonon density wave) provoked by a heat pulse, analogous to ordinary sound in a fluid, which is pressure wave propagation. The propagation of a heat pulse in the hydrodynamic regime is much different from those in diffusive or ballistic regimes as shown in Fig. 1c,d . The pulse in the hydrodynamic regime is transmitted by many N-scatterings [4] , [9] , [44] , [45] , whereas the pulse in the diffusive regime is largely damped by R-scattering and cannot propagate. The transmission of a heat pulse can also be observed in ballistic transport, but the sample size is limited to below phonon mean free path. Therefore, the phenomenon of second sound can provide a unique way to transmit a heat pulse without leaving a temperature trace behind the wave front in a sample larger than phonon mean free path. It is important to note that second sound is different from acoustic sound in a solid because the former is a phonon density wave, which is a collective motion of phonons in a wide spectrum maintained by many N-scattering processes, whereas the latter is just ballistic transport of extremely long-wavelength phonons. The required conditions on temperature and sample size for second sound are determined from the relative strength between N-scattering and momentum-destroying scatterings [26] . The frequency of second sound or the inverse of a pulse duration time ( Ω ) should be larger than the combined rate of U-scattering, isotope scattering and boundary scattering ( τ RB −1 , hereafter RB-scattering refers to U-scattering, isotope scattering and boundary scattering combined), but smaller than the N-scattering rate ( τ N −1 ). The former condition minimizes damping due to RB-scatterings. In particular, boundary scattering is not desirable for second sound, while it provides an important feature of phonon Poiseuille flow. The latter condition in equation (3) allows enough time to form a well-defined phonon density pulse. Otherwise, the phonon excitation would be randomized by N-scattering and would not form a pulse, analogous to the situation where an ordinary sound in a fluid is strongly damped when the sound frequency is high and comparable to the rate of scattering between molecules [46] . In Fig. 4a,b , we show a wide range of second sound frequencies in graphene below 100 K. The frequency range of second sound in graphene becomes narrow on the inclusion of isotope and boundary scatterings, but is still considerable when the sample is larger than 100 μm and isotope content is less than 0.1%. However, the frequency range of second sound in diamond does not exist for the given conditions since equation (3) cannot be satisfied. Shown in Fig. 4c,d are contour plots of second sound frequency range for various sample sizes, isotope contents and temperature conditions. In the same examined range of sample sizes, isotope concentration and temperature for Fig. 4c,d , we found that second sound is not possible at all in diamond. Similar to phonon Poiseuille flow, the main difference between graphene and diamond is attributable to the extremely strong N-scattering compared with R-scattering in graphene. 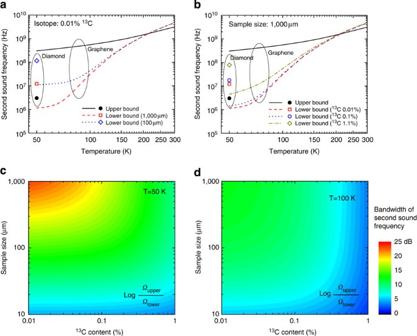Figure 4: The possible frequency ranges of second sound in graphene and diamond. The lower bound, calculated from momentum-destroying scattering rates, is required to minimize damping effects from the momentum-destroying scattering processes. The upper bound, calculated from N-scattering rates, is for phonons to maintain a well-defined heat pulse through many N-scattering processes. (a) The content of isotope13C is fixed at 0.01 %. (b) The sample size is fixed at 1,000 μm. (c,d) Contour plots of second sound frequency range in graphene with respect to sample size and isotope content for 50 and 100 K, respectively. The second sound frequency range is defined asΩupper/Ωlower, whereΩupperandΩlowerare the upper and lower bounds of second sound frequency, respectively. The frequency range is plotted on a log scale in the contour plots. Second sound in diamond is not possible in the given range of temperature, sample size and isotope content. Figure 4: The possible frequency ranges of second sound in graphene and diamond. The lower bound, calculated from momentum-destroying scattering rates, is required to minimize damping effects from the momentum-destroying scattering processes. The upper bound, calculated from N-scattering rates, is for phonons to maintain a well-defined heat pulse through many N-scattering processes. ( a ) The content of isotope 13 C is fixed at 0.01 %. ( b ) The sample size is fixed at 1,000 μm. ( c , d ) Contour plots of second sound frequency range in graphene with respect to sample size and isotope content for 50 and 100 K, respectively. The second sound frequency range is defined as Ω upper / Ω lower , where Ω upper and Ω lower are the upper and lower bounds of second sound frequency, respectively. The frequency range is plotted on a log scale in the contour plots. Second sound in diamond is not possible in the given range of temperature, sample size and isotope content. Full size image The second sound has been experimentally confirmed by measuring transient temperature response after applying a heat pulse [4] , [9] , [44] , [45] , [47] . One can apply a heat pulse at one side of a sample and measure temperature change with respect to time, d T /d t , at the other side of the sample. If a clear peak in d T /d t is observed, it can be attributed to either ballistic or hydrodynamic transport. The second sound peak can be distinguished from a ballistic pulse using the fact that the propagation of second sound is slower than the propagation of acoustic sound or ballistic phonon transport. For three-dimensional materials, it is theoretically estimated that the speed of second sound, v II , is where v I is the speed of acoustic sound in Debye model [2] , [48] , [49] . In past experiments, a clear peak in d T /d t was observed with a delay time that could be explained well with the theoretical prediction of the speed of second sound, . The second sound in graphene can be measured in a similar way as in the three-dimensional material cases. However, the speed of second sound cannot be estimated as because the Debye model is not valid for graphene due to the quadratic ZA branch. Instead of assuming a Debye model, we calculated the speed of second sound using the phonon dispersion determined from first principles. (see Methods for details) The calculated speed of second sound in graphene is plotted in Fig. 5a . In the figure, the speed of second sound ranges from 2,000 to 3,000 m s −1 and slightly increases with temperature. The dependence on temperature is because the group velocity of ZA phonon modes increases with frequency. At low temperatures where the most excited phonons are low-frequency phonons, the average group velocity is small, resulting in slower propagation of second sound than that of the high temperature cases. It would be interesting to see how the speed of second sound is compared with the speed of ballistic transport in graphene. In Fig. 5b , we compare the delay time of ballistic transport pulse and second sound in the heat pulse experiment mentioned above. The delay time of a ballistic transport pulse was calculated based on Landauer’s formalism [50] . (see Methods for details) In Fig. 5b , there is a significant broadening in the ballistic transport pulse because the group velocity of ZA phonon modes largely depends on frequency. In addition, the ballistic heat pulse becomes faster at higher temperature because high frequency phonons with large group velocity are excited. We also plot the delay time of second sound based on the calculated speed of second sound in Fig. 5a . The delay time of second sound is around three times longer than that of the peak of ballistic heat pulse. The difference in delay time by three times, together with the estimated speed of second sound, can be used to separate second sound signal from ballistic heat pulse. 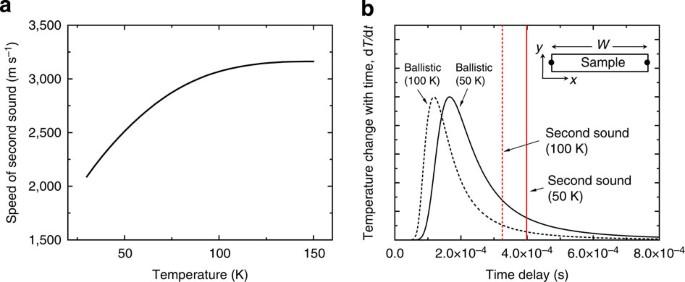Figure 5: The propagation speed of second sound. (a) The speed of second sound in graphene with respect to temperature (b) Comparison between the delay times by ballistic transport and by second sound propagation in the heat pulse experiment. The delay time is per distance between the source and the sensor,W, in (m). The inset illustrates the configuration of the sample with a point heat source and a point heat sensor for observing second sound. Figure 5: The propagation speed of second sound. ( a ) The speed of second sound in graphene with respect to temperature ( b ) Comparison between the delay times by ballistic transport and by second sound propagation in the heat pulse experiment. The delay time is per distance between the source and the sensor, W , in (m). The inset illustrates the configuration of the sample with a point heat source and a point heat sensor for observing second sound. Full size image The large contrast between graphene and diamond regarding hydrodynamic transport indicates that there are more reasons for the significant hydrodynamic transport in graphene, in addition to its large Debye temperature. Here we show that extremely large anharmonicity and density-of-states of long-wavelength ZA phonons, both originating from two-dimensional characteristics, are responsible for the significant hydrodynamic transport. The strong three-phonon scattering in graphene reflects a large phonon mode anharmonicity. The mode Grüneisen parameters give a measure of this anharmonicity [51] , and their magnitudes become large as wavelength increases ( Fig. 6a ). The extremely large magnitude of the Grüneisen parameters of the ZA modes near the zone centre is a characteristic of two-dimensional materials as explained by elasticity theory [52] . The elasticity theory predicts the divergence of the mode Grüneisen parameter, as γ q ~−1/| q | 2 where γ q is a mode Grüneisen parameter at wavevector, q . The actual divergence, however, is prevented by the strong phonon renormalization effect or any in-plane strain that stiffens the ZA phonon dispersion very near the zone centre [52] , [53] , [54] . In general, at large wavelengths, the three-phonon scattering processes are dominated by N-scattering since U-processes by definition require large-wavelength phonons. In particular, due to its large Debye temperature, phonons in graphene are predominantly populated in the large-wavelength region, further making N-scattering much stronger than U-scattering. This strong N-scattering is consistent with the behaviour of the mode Grüneisen parameters for ZA phonons in Fig. 6a and is confirmed in Fig. 3b,c , and also has been previously reported [19] , [55] . 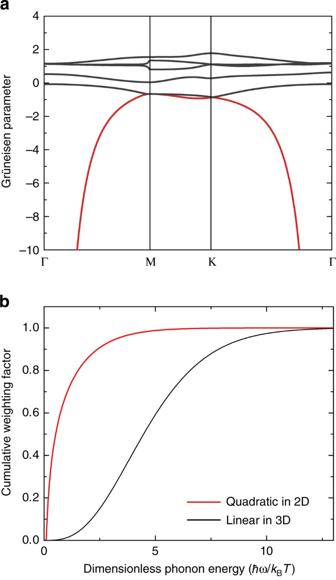Figure 6: The two-dimensional features of phonon modes in graphene responsible for the significant hydrodynamic phonon transport. (a) The mode Grüneisen parameter showing the large anharmonicity of long-wavelength ZA phonon modes. The red line corresponds to the ZA branch. (b) Cumulative weighting factors for averaging scattering rates for quadratic dispersion in two-dimensional materials and linear dispersion in three-dimensional materials. Figure 6: The two-dimensional features of phonon modes in graphene responsible for the significant hydrodynamic phonon transport. ( a ) The mode Grüneisen parameter showing the large anharmonicity of long-wavelength ZA phonon modes. The red line corresponds to the ZA branch. ( b ) Cumulative weighting factors for averaging scattering rates for quadratic dispersion in two-dimensional materials and linear dispersion in three-dimensional materials. Full size image The large gap between N- and R-scattering rates in graphene shown in Fig. 3b,c is further highlighted when considering the frequency range that mostly contributes to thermal transport. The transport regime, such as hydrodynamic or diffusive, is determined by comparing average scattering rates of N- and R-process as seen in second sound. It is noteworthy that the frequency ranges largely contributing the average scattering rates are different for graphene and diamond, because of their differing phonon density-of-states. The density-of-states is a constant for the quadratic dispersion in two-dimensional materials, while it increases with the square of frequency for the linear dispersion in three-dimensional materials. Therefore, the density-of-states of low-frequency phonons in the former case is much larger than that of the latter case, implying that role of low-frequency phonons in graphene is very significant. In Fig. 6b , we present the cumulative weighting factor for averaging the scattering rates as a function of phonon frequency. (see Methods for the definition of the cumulative weighting factor.) The cumulative weighting factor shows that the frequency ranges that are important for the averaged scattering rate are very different for diamond and graphene. From Fig. 6b , low-frequency phonons are most important for the quadratic dispersion in two-dimensional materials, whereas mid-frequency phonons give a larger contribution for the linear dispersion in three-dimensional materials. The significant role of low-frequency phonons in graphene results in the robust hydrodynamic phonon transport since low-frequency phonons exhibit a larger gap between N- and R-scattering rates as shown in Fig. 3b,c . In conclusion, we predict the hydrodynamic phonon transport in suspended graphene that is clearly distinguishable from the usual diffusive or ballistic phonon transport. The significant hydrodynamic transport in graphene is attributed to two-dimensional features such as extremely large scattering rates for momentum conserving N-processes and large density-of-states of long-wavelength ZA phonons. The significant hydrodynamic phonon transport in graphene provides a new perspective beyond diffusive and ballistic transport pictures to understand thermal transport in two-dimensional materials. In this work, we have focused on the sub-room temperature range, where hydrodynamic transport dominates over diffusive transport, but the hydrodynamic transport is also important for room temperature cases. The phonon transport in graphene at room temperature cannot be solely described by the diffusion limit due to strong N-scattering [55] , and the hydrodynamic transport presented here indicates another limit one may need to consider to fully understand phonon transport in graphene at room temperature. In addition, the significant hydrodynamic features imply practical importance. For example, considering the importance of boundary scattering shown in phonon Poiseuille flow, thermal rectification would be achievable in a tapered graphene sheet. The fast thermal transport without damping featured in second sound also shows a potential usage of graphene as thermal interconnects or thermal signal transmitters. Phonon distribution function from first principles The second- and third-order force constants of graphene were calculated from the density functional perturbation theory [56] , [57] using the Quantum-Espresso package [58] . The pseudopotential contains 2 s 2 p 2 as valence states with the Perdew–Zunger exchange-correlation functional [59] . The calculated force constants were validated by comparing mode Grüneisen parameters as in previous studies [19] , [21] . (see Supplementary Fig. 2 ) The force constants of diamond were adopted from ref. 60 . The three-phonon scattering rates were calculated using perturbation theory [15] . The strong renormalization effect for long-wavelength ZA phonons in graphene was included by using phonon stiffening parameters from ref. 52 . For the isotope scattering calculation, the 13 C isotope was treated as a point defect [61] . Using the calculated three-phonon and phonon-isotope scattering rates, the linearized Peierls–Boltzmann equation was solved with the iterative method [16] for the distribution function under a temperature gradient. For calculating scattering rates and solving the Peierls–Boltzmann equation, the first Brillouin zone was sampled with 70 × 70 and 30 × 30 × 30 meshes for graphene and diamond, respectively. The condition for phonon Poiseuille flow If phonons exhibit the displaced distribution, the transport of all phonon modes can be described by a single parameter, the displacement. Exploiting this feature, the macroscopic momentum balance equation can be derived from the Peierls–Boltzmann equation by taking crystal momentum as a moment [26] , [62] . Assuming a two-dimensional material, the momentum balance equation is where v is a group velocity and isotropic phonon dispersion is assumed. The above equation contains inner products of the eigenstates of the N-scattering operator, |0› and |1›. The eigenstates, |0› and |1›, represent the deviation of phonon distribution due to the temperature variation in real space and to a drift velocity, respectively [25] . Both eigenstates are expressed as [13] , [25] where x is the dimensionless phonon frequency, ħω / k B T . The ϕ and θ represent normalization factors for each state and α denotes a direction. The a 0 ( x ) and a 1 ( x ) in equation (4) are weights of the two states in the actual distribution at position x in real space. The physical meanings of a 0 ( x ) and a 1 ( x ) are temperature and drift velocity, respectively. The detailed derivation and discussion can be found in refs 13 , 25 , 26 , 62 . Equation (4) was originally derived for isotropic and linear dispersion [13] , [26] , but then extended to general cases [62] . Equation (4) looks similar to the Stokes equation, which is the macroscopic momentum balance equation for molecules when there is no change in the drift velocity along the flow direction, and thus the inertia term in the Navier–Stokes equation is removed. The right-hand side shows momentum gain by the temperature gradient, analogous to the pressure gradient term in the Stokes equation. The first term on the left-hand side means momentum transfer by N-scattering, analogous to the viscous term in the Stokes equation. The second term on the left-hand side reflects the momentum loss by R-scattering and does not have any counterpart in the Stokes equation. Therefore, for phonon Poiseuille flow to occur, the viscous effect, ‹1| v 2 τ N |1› ∇ 2 , should be larger than the R-scattering effect, ‹1|τ R −1 |1›. To compare the strength of the first and the second terms on the left-hand side, we estimate the ∇ 2 operator as ( L /2) −2 , where L is a sample width. Then, the required condition for the viscous effect being larger than the R-scattering effect is Adding the condition for non-ballistic transport to the above gives, where v y is a group velocity along the sample width direction. The above criteria can be qualitatively understood with a random walk picture of phonon transport [26] , [35] . (see Supplementary Note 3 ) For phonon Poiseuille flow, second sound and spectral contribution to an averaged scattering rate calculations, we consider only the lowest phonon branches for graphene (ZA) and diamond (TA 1 ), respectively, since these branches carry most of heat at low temperature [55] , [63] , also as confirmed in our calculation. (see Supplementary Fig. 1 ) The condition for second sound The N- and RB-scattering rates calculated from first principles were averaged with the displaced state, |1› (refs 26 , 62 ). In the above expressions, we made a small modification from the original expression given by ref. 26 . Please see Supplementary Note 5 for details. Derivation of the speed of second sound The past studies theoretically estimated the speed of second sound in three-dimensional materials as where v I is the speed of acoustic sound in Debye model [2] , [48] , [49] . For graphene, however, its phonon dispersion cannot be described by Debye model because of the nearly quadratic ZA phonon branch. Here we derive the wave equation for second sound from the Peierls–Boltzmann equation for arbitrary phonon dispersion cases to estimate the speed of second sound. We assume that R-scattering is negligibly weak and thus crystal momentum is approximately conserved. We start from the Peierls–Boltzmann transport equation for phonon transport. where the right-hand side represents the change in the phonon distribution due to scattering. Taking energy and crystal momentum along the flow direction as a moment leads to the macroscopic equations for energy and momentum balance, respectively. where λ is the phonon polarization. The right-hand side of equation (13) is zero because energy is always conserved on scatterings. The right-hand side of equation (14) is also zero because here we assume R-scattering is negligibly weak and thus crystal momentum is conserved. The actual phonon distribution ( N ) under very weak R-scattering can be approximated as the displaced distribution function as we confirmed in Fig. 2 . The displaced distribution can be linearized because the displacement in phonon distribution has a very small value: In addition, we can neglect higher-order terms associated with the small displacement ( u x ) in equations (13) and (14). The resulting equations are Taking the time derivative of equation (16) and the spatial derivative of equation (17), and then subtracting these two equations result in the hyperbolic wave equation for second sound. where v II represents the speed of second sound and can be expressed as The above expression can be simplified using the notation, |0› and |1›. Applying the Debye model for three-dimensional materials into equation (20) gives as previously derived [2] , [48] , [49] . For graphene, we calculate the speed of second sound using equation (20) and the phonon dispersion of ZA branch from first principles. We also calculated the speed of second sound by including all three acoustic branches for the inner products in equation (20), but the speed of second sound is almost same as that by including only ZA branch. Delay time of ballistic heat pulse Unlike other three-dimensional materials, the speed of ballistic transport in graphene cannot be represented by a single value of the speed of acoustic sound because of the quadratic ZA phonon branch. The group velocity, which largely depends on phonon frequency, can cause a significant broadening in a ballistic heat pulse. To take account of this effect, we suppose an experiment for observing second sound, similar to the past experiments for three-dimensional materials [4] , [9] , [45] , [47] . Suppose we have a rectangular shape graphene sheet with a point heat source at the left edge and a point thermal sensor at the right edge, as illustrated in the inset of Fig. 5b . At t =0, a heat pulse is generated at the point source with a delta function profile with respect to time. Assuming that all phonon modes transport ballistically, then the temperature change at the sensor can be expressed using the Landauer’s formalism [50] . where W is a distance between the source and the sensor. The Δ T is a temperature difference between the source and the sensor at t =0 + . The delta function of v y is included because phonon modes propagating with an oblique angle to the x direction cannot contribute to the ballistic thermal transport between the point source and the point sensor. This constraint prevents any additional broadening of the ballistic heat pulse from the finite size of the source and the sensor. In the actual cases where the source and the sensor have finite size, the temperature signal should be broader than that given by equation (22). Using equation (22) and phonon dispersion of ZA modes from first principles, we plot the temperature signal in ballistic transport in Fig. 5b . Spectral contribution to the averaged scattering rate In the macroscopic transport equation like equation (4), the scattering rate is averaged using the displaced state,|1›. Similarly, we define the cumulative weighting factor for averaging scattering rate as where ξ is one for quadratic dispersion in two-dimensional materials and four for linear dispersion in three-dimensional materials. The values of ξ can be derived from the definition of the state, |1›, in equations (5) and (6) by assuming isotropic phonon dispersion. In fact, for the case of perfectly quadratic dispersion in two-dimensional materials ( ξ =1), the low-frequency contribution to the averaged scattering rate diverges as frequency approaches zero. Such a singular behaviour is prevented by phonon stiffening from the renormalization effect. The spectral contribution in Fig. 6b includes the renormalization effect by using phonon stiffening parameters given in ref. 52 . How to cite this article: Lee, S. et al . Hydrodynamic phonon transport in suspended graphene. Nat. Commun. 6:6290 doi: 10.1038/ncomms7290 (2015).